Late-stage C–H functionalization of complex alkaloids and drug molecules via intermolecular rhodium-carbenoid insertion Alkaloids constitute a large family of natural products possessing diverse biological properties. Their unique and complex structures have inspired numerous innovations in synthetic chemistry. In the realm of late-stage C–H functionalization, alkaloids remain a significant challenge due to the presence of the basic amine and a variety of other functional groups. Herein we report the first examples of dirhodium(II)-catalysed intermolecular C–H insertion into complex natural products containing nucleophilic tertiary amines to generate a C–C bond. The application to a diverse range of alkaloids and drug molecules demonstrates remarkable chemoselectivity and predictable regioselectivity. The capacity for late-stage diversification is highlighted in the catalyst-controlled selective functionalizations of the alkaloid brucine. The remarkable selectivity observed, particularly for site-specific C–H insertion at N -methyl functionalities, offers utility in a range of applications where efficient installation of synthetic handles on complex alkaloids is desired. The decline in the number of new drug approvals in recent years despite high levels of R&D investment has spurred a number of alternative approaches towards drug discovery within the pharmaceutical industry [1] . This includes a resurgence in phenotypic screens, and along with that a renewed interest in exploiting the unique structural diversity of natural products to modulate disease-relevant processes [2] , [3] , [4] , [5] . Drug-discovery efforts around natural product optimization have been underexplored, owing in part to the synthetic challenge of effecting useful modifications in the face of structural complexity and diverse functionality. Advances in synthetic methodology are therefore essential to enable progression of natural product hits of compelling phenotype into suitable probes for elucidating mechanism of action and towards the development of new therapeutics [6] , [7] . C–H functionalization is one such approach that has the potential to revolutionize how complex organic molecules, such as natural products, are made through the ability to selectively and efficiently transform C–H bonds in a predictable manner under mild conditions. Over the last two decades, the field of C–H functionalization has experienced explosive growth, and a number of highly effective transformations have been developed. Many compelling examples have been reported on the utilization of C–H functionalization as key strategic reactions in total synthesis, illustrating novel retrosynthetic analysis and step-economical synthesis [8] , [9] , [10] , [11] , [12] , [13] . In recent years, considerable efforts have been expended on the late-stage C–H functionalization of biologically compelling natural products and drug-like molecules [14] , [15] , [16] , [17] , [18] , [19] , [20] , [21] , [22] . This has been challenging, because although the pace of advances in C–H functionalization has been impressive, in many instances the new methodology is limited to a narrow range of substrates and functional groups. Many of the most effective C–H functionalization processes rely on the use of directing groups, which need to be introduced and then removed [23] . Consequently, the late-stage C–H functionalization examples demonstrated to date often use rather specialized substrates and are of limited generality. Our aim is to select structurally complex molecules of compelling biological activity and then attempt to devise approaches to execute site-selective modification of C–H bonds in such compounds bearing multiple functional groups. The overarching goal is to establish a toolkit of reactions and reagents amenable to effecting functionalizations on a variety of complex molecules in a relatively predictive and selective manner for broad application. Alkaloids represent an extremely challenging class of natural products for direct C–H functionalization, because they typically contain a basic amine and a variety of other reactive functionality. In particular, a basic amine can impede many C–H-activation methodologies, as the nitrogen functionality may coordinate to and poison the catalyst [24] , [25] , [26] or generate undesirable side reactions [27] , [28] . Only a few examples of selective oxidation [29] , [30] or C–H amination of alkaloid derivatives have been reported, although in the case of the latter aza-ylide products are also formed and in many cases are the exclusive product [27] . One of the most effective methods for site-selective C–H functionalization, without resorting to the use of directing groups, has been the C–H insertion chemistry of rhodium-bound donor/acceptor carbenes [31] . Herein we demonstrate for the first time that such highly reactive intermediates are indeed capable of undergoing site-selective C–H functionalization of a range of complex alkaloids and drug molecules possessing a tertiary amine. We show that our effective strategy enables C–H functionalization at methyl, methylene or methine sites proximal to the basic amine, with little to no aza-ylide formation. This study constitutes a proof of concept that we envision can be readily extended to a wide range of applications, where efficient installation of synthetic handles on complex alkaloids may find utility. For instance, such a paradigm would be expected to greatly facilitate the ability to derivatize payloads for attachment to monoclonal antibodies for antibody–drug conjugate systems [32] , and in probe design for target identification or mechanism of action studies in a chemical genetics context [27] , [33] . Rhodium-carbenoid-mediated C–H functionalization of brucine Brucine ( 1 ) is a readily available complex natural product, which contains 22 C–H bonds in different chemical environments. The presence of two doubly activated allylic sites, a complex multi-ring architecture, a lactam functionality, an electron-rich phenyl ring, methyl ethers, as well as a basic tertiary amine offered a challenging target on which to commence these studies. A metal-free carbene approach to derivatize brucine was recently reported, which yielded a ring-expanded product through formation of an aza-ylide species followed by a [1,2]-Stevens rearrangement [34] . Indeed, the use of metallocarbenoids to access an aza-ylide intermediate followed by ring expansion has been widely described [35] , [36] , [37] . Interested in effecting C–H insertions via a carbenoid approach, we were intrigued as to whether the presence of a suitable rhodium catalyst and appropriate temperature might influence the nature of the reaction with brucine, allowing for C–H insertion over aza-ylide formation or catalyst poisoning, despite the presence of the nucleophilic amine. To the best of our knowledge, the ability to effect such chemistry on substrates possessing a tertiary amine, especially in structurally complex alkaloids, has not been previously reported [31] , [38] . As illustrated in Fig. 1a , we first compared the influence of a dirhodium catalyst in contrast to a metal-free system. Brucine was treated with excess methyl- p -bromophenyl diazoacetate ( 2 ) in the presence or absence of the well-established carbenoid C–H insertion catalyst Rh 2 ( S -DOSP) 4 (ref. 31 ) in trifluorotoluene at 83 °C (oil bath temperature). We observed that the Rh 2 ( S -DOSP) 4 -catalysed reaction provided C–H insertion product 3 in 20% yield as a single diastereomer, in addition to the expected Stevens rearrangement product 4 in 58% yield with 1.2:1 diastereomeric ratio (dr). When the same reaction was carried out in the absence of Rh 2 ( S -DOSP) 4 , formation of 3 and 4 was not observed, strongly suggesting that effective functionalization of brucine was mediated via the dirhodium catalyst. Attempting the Rh 2 ( S -DOSP) 4 -catalysed reaction at ambient temperature in either dichloromethane or trifluorotoluene failed to afford compound 3 or 4 . The differential outcome observed when conducting the reaction at room temperature as opposed to 83 °C led us to rationalize that a higher temperature enables a more rapid kinetic dissociation of the amine from the dirhodium catalyst. No longer incapacitated, the catalyst is free to effect diazo decomposition and carbenoid formation. 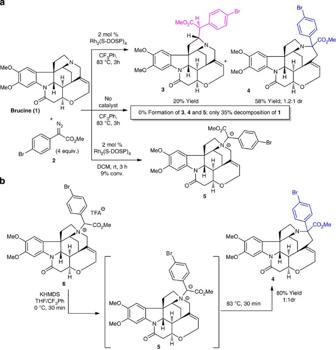Figure 1: Donor/acceptor rhodium-carbenoid-mediated functionalization of brucine (1). (a) Investigations into the role of the catalyst and temperature. (b) Control experiment provided mechanistic insights for the formation of C–H insertion product3. Conversion, yield and dr were determined by1H NMR with addition of 4-dimethylaminopyridine (DMAP) after work-up as an internal standard. rt, room temperature. Figure 1: Donor/acceptor rhodium-carbenoid-mediated functionalization of brucine (1). ( a ) Investigations into the role of the catalyst and temperature. ( b ) Control experiment provided mechanistic insights for the formation of C–H insertion product 3 . Conversion, yield and dr were determined by 1 H NMR with addition of 4-dimethylaminopyridine (DMAP) after work-up as an internal standard. rt, room temperature. Full size image Control experiment Having isolated aza-ylide 5 , we postulated whether formation of C–H insertion product 3 actually proceeded through a non-rhodium-bound ylide intermediate (as proposed in the formation of 4 ) [34] aided by thermal activation. Accordingly, a control experiment was conducted as presented in Fig. 1b . Aza-ylide 5 was alternatively prepared in situ through deprotonation of the corresponding trifluoroacetate salt 6 at 0 °C. The reaction was heated to 83 °C in a pressure vessel for 30 min, yielding exclusively [1,2]-Stevens rearrangement product 4 in 1:1 dr. Since C–H insertion product 3 was not observed, it suggests that ylide formation and carbenoid C–H insertion proceed through different reaction pathways. Indeed, we speculate that product 3 is formed via direct C–H insertion induced by the metal carbene [39] , [40] . This being the case, it is remarkable that 3 is the sole C–H insertion product observed from a molecule that has numerous potential sites for C–H functionalization. The subtle balance between electronic, steric and stereoelectronic effects can often result in exquisite regiocontrol in the C–H functionalization reactions of donor/acceptor rhodium carbenes [31] , but such control has not been previously demonstrated with such a complex substrate. Influence of dirhodium catalysts The electrophilicity and steric environment of the metallocarbenoids can be affected by the nature of the catalyst [31] . Hence, we were eager to explore what influence various dirhodium catalysts would have on the site selectivity of the reaction ( Table 1 ). The bulky dirhodium catalyst Rh 2 (TPA) 4 promoted formation of the C–H insertion product, giving 3 in 50% yield as a single diastereomer. Subsequent investigations into other achiral rhodium catalysts ( Table 1 , entries 2–5) revealed that Rh 2 (TPA) 4 is the most effective catalyst for carbenoid-mediated C–H insertion. In addition, the formation of Stevens rearrangement product 4 is a competing pathway for which the chemoselectivity between the formation of compounds 3 and 4 is catalyst dependent. Furthermore, the two enantiomers of chiral catalysts afforded different results. For example, only the use of the S -enantiomer of the DOSP ligand allowed for C–H insertion ( Table 1 , entries 7 and 8). A most unexpected result was obtained with the very bulky chiral catalyst Rh 2 (BTPCP) 4 refs 41 , 42 . Under the standard reaction conditions, the Rh 2 (BTPCP) 4 -catalysed reactions suffered very poor conversion, irrespective of whether the R- or S -enantiomer of the catalyst was used ( Table 1 , entries 11 and 12). Careful 1 H nuclear magnetic resonance (NMR) analysis of the crude reaction mixture revealed an alternative C–H insertion product ( 7 ) had been generated in low yield with Rh 2 ( S -BTPCP) 4 . Increasing the catalyst loading of Rh 2 ( S -BTPCP) 4 to 20 mol% afforded compound 7 in 39% yield as a single diastereomer, albeit with moderate conversion ( Fig. 2a ). Extensive one- and two-dimensional NMR experiments confirmed that this new compound 7 was generated through C–H insertion into the tertiary C–H bond adjacent to the amine. The ability for Rh 2 ( S -BTPCP) 4 to enable selective C–H insertion at the methine position is unexpected, because a bulky catalyst should generally favour functionalization of a less-sterically encumbered C–H bond [42] . The catalyst screen reveals that one can manipulate the favoured site for functionalization in a catalyst-controlled manner, allowing one to rapidly probe three alternative sites on a complex molecule ( Fig. 2a ). Table 1 Influence of dirhodium catalyst on C–H carbene insertion of brucine (1). 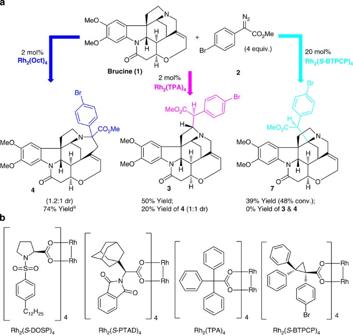Figure 2: Optimization of rhodium-catalysed C–H carbene insertion of brucine (1). (a) Catalyst influence on site-selective C–H functionalization of brucine (1). (b) Structures of dirhodium catalysts. Conversion, yield and dr were determined by1H NMR analysis with addition of 4-dimethylaminopyridine after work-up as an internal standard, unless otherwise specified.aIsolated yield. Full size table Figure 2: Optimization of rhodium-catalysed C–H carbene insertion of brucine (1). ( a ) Catalyst influence on site-selective C–H functionalization of brucine ( 1 ). ( b ) Structures of dirhodium catalysts. Conversion, yield and dr were determined by 1 H NMR analysis with addition of 4-dimethylaminopyridine after work-up as an internal standard, unless otherwise specified. a Isolated yield. Full size image Diazo scope Studies with a small set of aryldiazoacetates of distinct electronic properties indicate that the nature of the carbenoid also plays a role in the chemoselectivity of the rhodium-carbenoid insertion ( Table 2 , entries 1–3). Donor/acceptor carbenoids bearing electron-deficient aryl substituents favoured C–H insertion product 9 over aza-ylide formation ( Table 2 , entries 1 and 3), whereas an electron-donating substituent provides a less-electrophilic rhodium-carbenoid for which exclusive formation of ring-expanded product 10 was observed ( Table 2 , entry 2). Reaction with methyl diazomalonate ( 8c ) or ethyl diazoacetate ( 8d ) failed to generate any C–H insertion or Stevens rearrangement product ( Table 2 , entries 4 and 5), suggesting the importance of the donor group in the efficiency of intermolecular C–H insertion reactions under these conditions. Table 2 Influence of diazo reagents on rhodium-catalysed carbene insertion of brucine (1). Full size table C–H functionalization of securinine To explore reaction generality, we applied the Rh 2 (TPA) 4 -mediated approach to other structurally complex alkaloids and tertiary amine-containing drug molecules ( Figs 3 and 4 ). The GABA A antagonist securinine ( 12 ) is a tricyclic alkaloid possessing two olefins in conjugation with a lactone functionality, in addition to the tertiary amine ( Fig. 3a ). Treatment of 12 with methyl- p -bromophenyl diazoacetate ( 2 ) and Rh 2 (TPA) 4 in trifluorotoluene at 83 °C selectively gave C–H insertion product 13 (44% yield, 2.2:1 dr), with no competing cyclopropanation at either olefin [43] . Furthermore, although securinine contains four C–H bonds adjacent to the amine (two methine and two diastereotopic methylene in nature), only a single methylene C–H bond undergoes carbene insertion. Unlike the case of brucine in which substrate control afforded a highly diastereoselective C–H insertion product, with securinine the diastereoselectivity was rather moderate, and was influenced by the dirhodium catalyst itself ( Fig. 3a ). 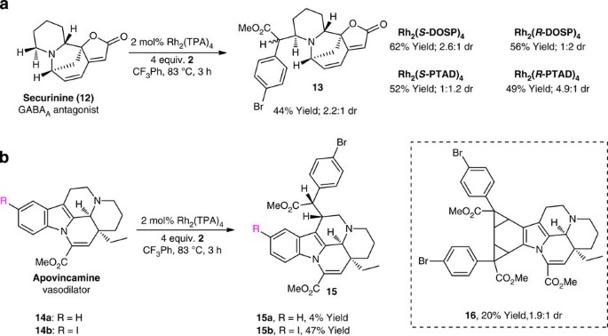Figure 3: Rhodium-catalysed C–H insertion of alkaloids securinine and apovincamine. (a) Diastereoselective C–H carbene insertion is achieved by using chiral rhodium catalysts. (b) Introduction of steric hindrance could protect electron-rich aromatic rings from cyclopropanation and enable desired C–H insertion. Yield and dr were determined by1H NMR analysis with addition of 4-dimethylaminopyridine after work-up as an internal standard, unless otherwise specified. Figure 3: Rhodium-catalysed C–H insertion of alkaloids securinine and apovincamine. ( a ) Diastereoselective C–H carbene insertion is achieved by using chiral rhodium catalysts. ( b ) Introduction of steric hindrance could protect electron-rich aromatic rings from cyclopropanation and enable desired C–H insertion. Yield and dr were determined by 1 H NMR analysis with addition of 4-dimethylaminopyridine after work-up as an internal standard, unless otherwise specified. 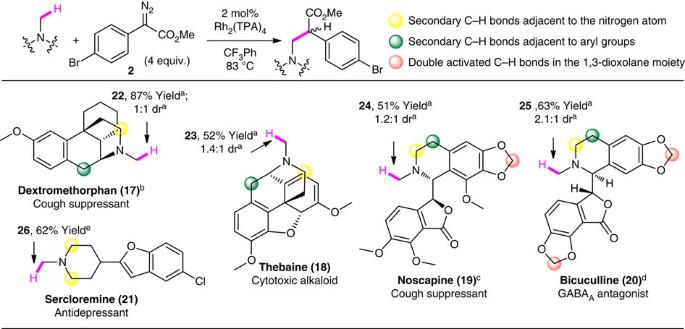Figure 4: C–H insertion inN-methyl-containing natural products and drug molecules. aYield and dr were determined by1H NMR with 4-dimethylaminopyridine as an internal standard.bReaction was carried out in dichloromethane under room temperature.cReaction was carried out with 0.5 equiv. of2in dichloromethane at room temperature (54% recovered SM).dReaction was carried out with 0.5 equiv. of2(52% recovered SM).eIsolated yield. Full size image Figure 4: C–H insertion in N -methyl-containing natural products and drug molecules. a Yield and dr were determined by 1 H NMR with 4-dimethylaminopyridine as an internal standard. b Reaction was carried out in dichloromethane under room temperature. c Reaction was carried out with 0.5 equiv. of 2 in dichloromethane at room temperature (54% recovered SM). d Reaction was carried out with 0.5 equiv. of 2 (52% recovered SM). e Isolated yield. Full size image C–H functionalization of apovincamine Further application of this method to apovincamine ( 14a ) led to bis-cyclopropanation of the electron-rich indole ring 16, with only minimal formation of the C–H insertion product ( Fig. 3b ) [44] . Attempts with other dirhodium catalysts provided similar reaction outcomes. It is well established that aromatic rings are sterically protected from reaction with rhodium donor/acceptor carbenoids when they are at least 1,4-disubstituted [45] . Accordingly, the iodinated apovincamine analogue 14b was prepared and evaluated in the reaction, and in this instance the C–H insertion product 15b was obtained in improved yield (47% yield) as a single diastereomer. Although 14b contains one methine and four methylene C–H bonds adjacent to the amine, the C–H insertion occurred selectively at the benzylic methylene site rather than alpha to the amine. Previously, it has been reported that benzylic C–H bonds are also favourable sites for C–H insertion, due to the capacity of π-systems to stabilize the neighbouring buildup of positive charge in the transition state [46] . Selective N -methyl C–H insertion C–H functionalization induced by dirhodium-bound donor/acceptor carbenoids has been shown to be initiated by a hydride transfer event, and sites that are capable of stabilizing positive charge buildup at carbon are electronically favoured [40] . However, the general order of reactivity of C–H bonds in competition reactions is typically methine~methylene>methyl, because although tertiary sites are electronically most activated, donor/acceptor carbenoids are sterically very demanding [31] . In the alkaloids studied so far the reactions have been remarkably site selective, suggesting that the majority of electronically activated methine and methylene sites in these alkaloids are sterically inaccessible. Therefore, we chose to explore the reactions of alkaloids containing N -methyl groups. Functionalization of electronically activated methyl C–H bonds has been observed, but only a few examples of C–H insertion into methyl C–H bonds in the presence of activated methylene and/or methine C–H bonds have been reported [42] , [47] , [48] , [49] , and none of those feature a basic amine. We found for alkaloids possessing an N -Me functionality, the most favoured product in each case arose from C–H insertion into the said N -methyl group ( Fig. 4 ). With dextromethorphan ( 17 ), for example, carbene insertion at the N -methyl C–H bond was the most favoured product despite methylene sites adjacent to the nitrogen atom and the phenyl ring. It is worth noting that no insertion was observed at the accessible methyl ether site. Indeed, C–H insertion at the N -methyl site was such a favoured pathway that we were able to effect the reaction at room temperature affording 87% yield of C–H insertion product (1:1 dr), with complete conversion of 17 . The structurally related yet more elaborate thebaine ( 18 ) smoothly underwent C–H insertion at the N -methyl site (52%, 1.4:1 dr), without any competing reactivity despite the electron-rich aryl group and the 1,3-diene functionality. It appears that regardless of conformation or neighbouring functionalities, in all systems explored the donor/acceptor carbenoid derived from 2 selectively inserts into the primary C–H bond adjacent to nitrogen. In addition, the apparent ease of insertion into the N -methyl group enables some reactions to be conducted at room temperature, with diazo 2 used as the limiting reagent, as was the case with noscapine ( 19 ), although the structurally related bicuculline ( 20 ) required more forcing conditions. Generally, the diastereoselectivity of the Rh 2 (TPA) 4 -mediated N -methyl insertion reactions afforded diastereomeric ratios in the 1:1-2:1 range, and the application of chiral dirhodium catalysts failed to improve on this ( Table 3 ). Sercloremine ( 21 ) represents an interesting substrate in that its relatively simple structure suggests little potential for steric differentiation between the methylene sites and the terminal methyl site adjacent to the amine, however, the N -methyl C–H insertion product is again exclusively formed in 62% yield. It should be noted that Stevens-type rearrangement products were not observed in any of the N -methyl-containing systems explored in this study and presumably is no longer a competing pathway. It is likely that the ease of accessibility the primary C–H bond offers has a significant impact on the site-selectivity of this reaction. Table 3 Chiral dirhodium catalysts screen using bicuculline (20) as a substrate. Full size table We have successfully devised and implemented an effective strategy for non-directed C–H functionalization of nucleophilic tertiary amine-containing complex natural products and drug molecules. We demonstrate that these traditionally challenging substrates are capable of undergoing rhodium-catalysed C–H insertion reactions to selectively install a new C–C bond. The methods we describe are effectively implemented on a diverse set of alkaloids possessing a wide variety of architectures, functionalities and potentially reactive sites. The use of donor/acceptor carbenoids is the key to our ability to achieve such remarkable chemoselectivity and predictable regioselectivity. In addition, our approach obviates the challenging issue of undesired aza-ylide formation commonly observed with carbenoids in the presence of basic nitrogen-containing substrates, and in doing so the work significantly expands and enables the scope of this field [27] . The highly efficient generation of three distinct brucine derivatives in a catalyst-controlled fashion ( Fig. 2a ), showcases the potential of this approach to offer late-stage diversification of complex molecules. It is worth noting that the site of C–H insertion is routinely in proximity to the amine moiety. We look upon this consistency, in particular the remarkable selectivity for C–H insertion into N -methyl-containing alkaloids, as a robust and highly predictable approach for site-specific functionalization of complex molecules, which could be applied late on in a synthetic route for direct derivatization adjacent to an amine, or for the introduction of a synthetic handle for use in bioconjugation strategies for chemical biology studies. Materials Materials were obtained from commercial suppliers and used as received, or prepared according to standard procedures, unless otherwise noted. Sercloremine ( 21 ) and apovincamine ( 14a ) were obtained from the Novartis compound archive. Methyl- p -bromophenyl diazoacetate ( 2 ) as well as its analogues 8a and 8b were synthesized according to a previously reported procedure [43] . All reactions were conducted under an inert atmosphere of dry nitrogen. Analytical thin-layer chromatography was performed on Kieselgel 60 F254 (250 μm silica gel) glass plates and compounds were visualized with ultraviolet light 254 nm). Flash column chromatography was performed using Kieselgel 60 (230–400 mesh) silica gel with ethyl acetate/hexanes as eluent, unless indicated otherwise. General spectroscopic methods 1 H NMR spectra were measured at 400 MHz on a Bruker Avance instrument and reported in parts per million ( δ , p.p.m.). Coupling constants ( J- values) were reported in Hertz (Hz), with multiplicity reported following usual convention: s=singlet, d=doublet, t=triplet, q=quartet, dd=doublet of doublets, m=multiplet and br=broad. The proton signal of the residual, non-deuterated solvent ( δ 7.26 for CHCl 3 ) was used as an internal reference for 1 H NMR spectra. 13 C NMR spectra were completely hetero-decoupled and measured at 100 MHz. Residual chloroform ( δ 77.23) was used as an internal reference. Preparative high-performance liquid chromatography was performed using Waters Autopurification system with a photodiode array detector. Preparative supercritical fluid chromatography was performed using a Thar (Waters) SFC 80 preparative system with a Waters 2489 UV/visible detector. All tested compounds were found to be >95% pure (unless stated otherwise) as determined by liquid chromatography-UV (LC-UV)/electrospray ionization (ESI)-mass spectrometry (MS), recorded using an Acquity G2 Xevo OTof mass spectrometer (accuracy <5 p.p.m.) with an electrospray ionization source and Acquity ultra performance liquid chromatograph (conditions: Acquity UPLC BEH C18 1.7 μm 2.1 × 50 mm column, solvent A: water+0.1% formic acid, solvent B: acetonitrile+0.1% formic acid, gradient: from 2 to 98% B in 4.4 min, 1.0 ml min −1 flow rate and 50 °C). Ammonium salts, which were generated in preparative high-performance liquid chromatography with trifluoroacetic acid or formic acid as a modifier, were converted to the corresponding free amine with 4 equiv. MP-carbonate (Biotage) in 0.1 M dichloromethane for 1 h at room temperature. 1 H NMR, 13 C NMR and high-resolution mass spectra (HRMS) are provided for all compounds. For NMR spectra and detailed analysis of NMR assignments, see Supplementary Figs 1–28 ; Supplementary Notes 1–5 , respectively. For supercritical fluid chromatography analysis and ion chromatography analysis of 6 see Supplementary Notes 6,7 . See Supplementary Methods for the characterization data of compounds not listed in this section. Synthesis of 3 An oven-dried 10 ml two-necked round-bottom flask fitted with a condenser was charged with brucine ( 1 ) (133.2 mg, 0.338 mmol) and Rh 2 (TPA) 4 (9.7 mg, 6.8 μmol) in degassed trifluorotoluene (3.0 ml) under a nitrogen atmosphere. A solution of methyl- p -bromophenyl diazoacetate ( 2 ) (345 mg, 1.35 mmol) in degassed trifluorotoluene (3.8 ml) was slowly added via a syringe pump over 1 h under nitrogen atmosphere at 83 °C (oil bath temperature). The mixture was stirred at this temperature for 2 h and then concentrated in vacuo . 1 H NMR analysis with addition of 5.0 mg 4-dimethylaminopyridine as an internal standard indicated 3 was obtained in 50% yield as a single diastereomer and 4 in 20% yield (1:1 dr). The resulting crude was then purified through flash column chromatography (0–50% EtOAc/heptane) twice to afford 3 as a white solid (92.9 mg, 44% isolated yield, Rf=0.04 in 50% EtOAc/heptane). To aid analysis, 3 was isolated as the corresponding TFA salt. 1 H NMR (400 MHz, chloroform- d ) δ 7.76 (s, 1H), 7.59 (d, J =8.0 Hz, 2H), 7.44 (d, J =8.0 Hz, 2H), 6.91 (s, 1H), 6.01 (t, J =4.0 Hz, 1H), 4.77 (br, 1H), 4.36 (d, J =8.0 Hz, 1H), 4.35 (m, 1H), 4.24 (dd, J =16.0, 8.0 Hz, 1H), 4.06 (d, J =12.0 Hz, 1H), 3.96–4.06 (m, 2H), 3.91 (s, 3H), 3.90 (s, 3H), 3.86 (d, J =16.0 Hz, 1H), 3.63 (s, 3H), 3.26 (br, 1H), 3.20 (dd, J =16.0, 8.0 Hz, 1H), 2.73 (dd, J =16.0, 4.0 Hz, 1H), 2.42–2.51 (m, 2H), 2.29 (t, J =16.0 Hz, 1H), 2.17 (d, J =16.0 Hz, 1H), 1.67 (d, J =16.0 Hz, 1H), 1.39 (dt, J =8.0, 4.0 Hz, 1H). 13 C NMR (100 MHz, chloroform- d ) δ 170.9, 169.2, 161.7 (CF 3 ), 150.7, 147.5, 135.9, 135.5, 133.2, 132.9, 132.7, 130.3, 124.1, 118.8, 105.1, 101.3, 76.9, 66.7, 64.2, 63.5, 59.7, 56.5, 53.2, 52.5, 52.0, 51.4, 47.1, 46.1, 42.1, 30.5, 25.6. HRMS (ESI-time of flight (TOF)) [M+H] + calculated for C 32 H 34 BrN 2 O 6 : 621.1600; found: 621.1575. LC-UV/ESI-MS retention time: 1.70 min. Purification of the crude reaction mixture also afforded 4 contaminated with small amount of impurity. A subsequent purification through flash column chromatography (0–50% EtOAc/heptane) provided the two diastereomers of 4 as separate compounds (24.2 mg, 11% isolated yield, Rf=0.30 in 50% EtOAc/heptane; 17.2 mg, 8% isolated yield, Rf=0.25 in 50% EtOAc/heptane). 4a , diastereomer 1: 1 H NMR (400 MHz, chloroform- d ) δ 7.82 (s, 1H), 7.54 (d, J =8.6 Hz, 2H), 7.40 (d, J =8.6 Hz, 2H), 6.72 (s, 1H), 5.86 (q, J =3.8 Hz, 1H), 4.38 (dd, J =16.4, 5.0 Hz, 1H), 4.27 (m 1H), 4.10 (dm, J =16.4 Hz, 1H), 3.98 (d, J =11.1 Hz, 1H), 3.94 (s, 1H), 3.90 (s, 3H), 3.89–3.85 (m, 4H), 3.63 (s, 3H), 3.33–3.22 (m, 1H), 3.03 (d, J =16.0 Hz, 1H), 2.97 (t, J =7.5 Hz, 1H), 2.93 (m, 2H), 2.83 (s, 1H), 2.00 (dt, J =16.0, 4.0 Hz, 1H), 1.96–1.81 (m, 2H), 1.60 (dt, J =8.0, 4.0 Hz, 1H), 1.41 (d, J =15.5 Hz, 1H). 13 C NMR (100 MHz, chloroform- d ) δ 173.3, 170.0, 149.4, 146.3, 142.8, 138.3, 135.9, 131.7, 128.8, 128.4, 123.8, 121.5, 105.9, 101.1, 75.8, 68.7, 65.2, 62.9, 59.6, 56.8, 56.4, 53.2, 53.1, 49.4, 48.3, 47.0, 42.4, 39.5, 35.3, 31.7. HRMS (ESI-TOF) [M+H] + calculated for C 32 H 34 BrN 2 O 6 : 621.1600; found: 621.1594. LC-UV/ESI-MS retention time: 2.88 min. 4b , diastereomer 2: 1 H NMR (400 MHz, chloroform- d ) δ 7.81 (s, 1H), 7.48 (d, J =8.2 Hz, 2H), 7.26 (br, 2H), 6.67 (s, 1H), 5.52 (s, 1H), 4.28–4.13 (m, 2H), 4.09 (d, J =10.4 Hz, 1H), 4.00 (dm, J =14.8 Hz, 1H), 3.94 (s, 3H), 3.90 (s, 3H), 3.89 (s, 3H), 3.68 (d, J =15.2 Hz, 1H), 3.46 (d, J =4.2 Hz, 1H), 3.10 (dd, J =16.2, 8.3 Hz, 1H), 2.96 (s, 1H), 2.88–2.59 (m, 3H), 2.50–2.29 (m, 2H), 2.07–1.95 (m, 1H), 1.75–1.61 (m, 2H), 1.43 (dt, J =10.5, 4.5 Hz, 1H). 13 C NMR (100 MHz, chloroform- d ) δ 173.9, 170.5, 149.1, 146.5, 142.9, 142.1, 136.6, 131.5, 128.3, 128.1 (br), 124.1, 121.6, 105.7, 101.2, 79.3, 68.5, 67.0, 64.5, 60.4, 56.8, 56.4, 53.0, 52.1, 49.1, 47.9, 45.8, 42.2, 40.8, 35.2, 29.3. HRMS (ESI-TOF) [M+H] + calculated for C 32 H 34 BrN 2 O 6 : 621.1600; found: 621.1600. LC-UV/ESI-MS retention time: 3.03 min. How to cite this article : He, J. et al. Late-stage C–H functionalization of complex alkaloids and drug molecules via intermolecular rhodium-carbenoid insertion. Nat. Commun. 6:5943 doi: 10.1038/ncomms6943 (2015).